BES1 is activated by EMS1-TPD1-SERK1/2-mediated signaling to control tapetum development inArabidopsis thaliana BES1 and BZR1 were originally identified as two key transcription factors specifically regulating brassinosteroid (BR)-mediated gene expression. They belong to a family consisting of six members, BES1, BZR1, BEH1, BEH2, BEH3, and BEH4. bes1 and bzr1 single mutants do not exhibit any characteristic BR phenotypes, suggesting functional redundancy of these proteins. Here, by generating higher order mutants, we show that a quintuple mutant is male sterile due to defects in tapetum and microsporocyte development in anthers. Our genetic and biochemical analyses demonstrate that BES1 family members also act as downstream transcription factors in the EMS1-TPD1-SERK1/2 pathway. Ectopic expression of both TPD1 and EMS1 in bri1-116 , a BR receptor null mutant, leads to the accumulation of non-phosphorylated, active BES1, similar to activation of BES1 by BRI1-BR-BAK1 signaling. These data suggest that two distinctive receptor-like kinase-mediated signaling pathways share BES1 family members as downstream transcription factors to regulate different aspects of plant development. Brassinosteroids are essential plant hormones regulating multiple processes during plant growth, development, and stress adaptations [1] , [2] , [3] , [4] . Brassinosteroids (BRs) are perceived by a cell surface RLK complex, including their major receptor BRASSINOSTEROID INSENSITIVE 1 (BRI1) and co-receptor BRI1-ASSOCIATED RECEPTOR KINASE 1 (BAK1) [5] , [6] , [7] , [8] . Upon the activation of BRI1 and BAK1 [9] , [10] , [11] , an intracellular signaling cascade can be subsequently initiated [12] , including releasing a negative regulator BRI1 KINASE INHIBITOR 1 (BKI1) from the plasma membrane-localized BRI1 and BAK1 complex [13] , [14] , [15] , and inactivating second negative regulator BRASSINOSTEROID INSENSITIVE 2 (BIN2) by a phosphatase BRI1 SUPPRESSOR 1 (BSU1) [12] , [16] , [17] , [18] , [19] . Inactivation of BIN2 can greatly induce the accumulation of non-phosphorylated forms of two transcription factors, BRI1 EMS SUPPRESSOR 1 (BES1) and BRASSINAZOLE RESISTANT 1 (BZR1), in the nucleus [20] , [21] , [22] , [23] , [24] . Activated BES1 and BZR1 can then mediate the expression of thousands of downstream responsive genes by either directly associating with the promoters of their target genes or via interacting with different types of transcription factors [25] , [26] , [27] . It has been believed that BES1 and BZR1 are essential transcription factors in the BR signaling pathway to regulate target gene expression [20] , [21] . Loss-of-function genetic data supporting the importance of BES1 family members in the BR signaling pathway, however, are not fully established [28] . To investigate the genetic significance of BES1 family members in the BR signaling pathway, we isolated single mutants for all BES1 family genes and generated double, triple and higher order mutants. Interestingly, our quintuple mutants showed a complete male sterile phenotype due to lack of pollen grains in its anthers, suggesting that BES1 family members are also involved in pollen generation. Pollen grains are produced by anthers, the upper part of the male reproductive organ called stamen. The development of anthers in Arabidopsis involves 14 artificially divided stages according to previous morphological and cellular studies [29] , [30] , [31] . Anther primordium, consisting of three layers L1, L2, and L3, emerges from floral meristem at stage 1. During stages 2–5, cells from these three layers divide and differentiate to produce a fundamental anther architecture with four lobes which are connected by L3-derived vascular tissues and are covered by L1-derived epidermis. At the meantime, L2-derived cells within each of the four lobes develop into microsporocytes at the center and three surrounding somatic cell layers including tapetum, middle layer, and endothecium from the inner to outer. At stages 6–12, microsporocytes initiate meiotic division to generate microspores that further develop into mature pollen grains. Then, mature pollen grains are released at stage 13 and anthers finally collapse at stage 14. During anther morphogenesis, cell-to-cell communications are critical to the coordinated development of L2-derived layers such as microsporocytes and their nurturing somatic layer, tapetum [30] . Previous studies indicated that microsporocytes and their precursor cells (sporogenous cells) guide tapetum formation and differentiation via an RLK-mediated transmembrane signaling pathway [32] , [33] , [34] . Sporogenous cells and microsporocytes secret TAPETUM DETERMINANT 1 (TPD1), a small cysteine-rich peptide ligand, which can bind to and activate its receptor and co-receptor, EXTRA MICROSPOROCYTES1/EXTRA SPOROGENOUS CELLS (EMS1/EXS) and SOMATIC EMBRYOGENESIS RECEPTOR-LIKE KINASES 1 and 2 (SERK1 and 2) [32] , [35] , [36] , [37] , [38] , [39] , [40] . EMS1 is mainly localized in the inner secondary parietal layer (precursor of tapetum) and tapetum during anther patterning [32] . Although recent studies suggested that carbonic anhydrases act as direct targets of EMS1 in regulating tapetal cell differentiation, how activated TPD1-EMS1/SERK1/2 complex triggers downstream response gene expression is not fully understood [41] . Here we demonstrate that BES1 family members play key roles in anther development. Anthers of a quintuple mutant, bes1-1 bzr1-1 beh1-1 beh3-1 beh4-1 ( qui-1 ), show an incompletely developed tapetum-like cell layer, which losses normal tapetum cell identity. In addition, qui-1 displays excessive microsporocytes, similar to what is observed in ems1 , tpd1 , serk1/2 mutant anthers. Gain-of-function point mutation of BES1 or BZR1 , bes1-D or bzr1-1D , can partially restore the tapetum identity and pollenless defects of ems1 , tpd1 , and serk1/2 . Consequently, the fertilities of these mutants are considerably recovered. Ectopic expression of TPD1 and EMS1 leads to significant accumulation of non-phosphorylated BES1. Our data reveal that BES1 family members are the downstream transcription factors of the TPD1-EMS1/SERK1/2 signaling pathway and they play an essential role in plant reproduction via regulating tapetum development. BES1 family members are required for pollen production BES1 and BZR1 are two well-characterized transcription factors originally identified as downstream components of the BR signal transduction [20] , [21] . Loss-of-function mutants of BES1 or BZR1 do not show typical BR-related defects. Phylogenic analysis indicated that BES1 and BZR1 belong to a six-member family, including BES1, BZR1, BEH1, BEH2, BEH3, and BEH4 (Supplementary Fig. 1 ). We therefore ordered T-DNA insertion lines for all of the BES1 family member genes from Arabidopsis Biological Resource Center (ABRC). Genotypic analyses confirmed the true T-DNA insertions for BES1 , BZR1 , BEH1 , BEH3 , and BEH4 , but not for BEH2 . These five T-DNA insertion lines were subsequently named as bes1-1 , bzr1-1 , beh1-1 , beh3-1 , and beh4-1 , respectively (Supplementary Fig. 2a ). RT-PCR analyses proved that bzr1-1 , beh1-1 , and beh3-1 are true null mutants, in which full-length mRNAs cannot be detected (Supplementary Fig. 2b ). Previous studies indicated that BES1 has two alternatively spliced transcripts, BES1-L and BES1-S [42] . In bes1-1 , the BES1-L transcript is completely eliminated, whereas the BES1-S transcript is still present (Supplementary Fig. 2b ). Therefore, bes1-1 is not a complete knockout line, even though it was demonstrated that BES1-L is more functionally important than BES1-S [42] . beh4-1 is actually a knockdown mutant but not a null mutant (Supplementary Fig. 2b ). All these single mutants did not show any growth defects. We then generated different combinations of double, triple, and quadruple mutants. Double, triple, and quadruple mutants generated from these T-DNA alleles did not display obvious phenotypes. A quintuple mutant, bes1-1 bzr1-1 beh1-1 beh3-1 beh4-1 ( qui-1 ) showed a complete sterile phenotype (Fig. 1a, b and Supplementary Fig. 3 ). Filaments of qui-1 are much shorter than that of wild type and fail to elongate (Fig. 1c, d ). Microscopic assays indicated that the sterility is caused by lack of pollen grains in the anthers of the quintuple mutant (Fig. 1e–h and Supplementary Fig. 3g–l ). To further confirm that the male sterility is caused by the inactivation of the five BES1 family genes, we introduced the genomic sequences of five genes, mostly driven by their own promoters, into qui-1 individually (Supplementary Fig. 4 ). Cloning of BEH3 promoter was unsuccessful after multiple trials due to unknown reasons. UBQ10 promoter was therefore used to drive the expression of BEH3 (Supplementary Fig. 4 ). All the transgenic plants obtained showed fully recovered pollen development and fertility (Supplementary Fig. 4 ). These results indicated that the male sterility of the qui-1 is solely caused by the inactivation or partially inactivation of five BES1 family genes. qui-1 is not a complete knockout line and it does not show any obvious vegetative growth defects besides its male sterility. Therefore, most of our subsequent analyses were performed by using qui-1 . Fig. 1 A quintuple mutant, bes1-1 bzr1-1 beh1-1 beh3-1 beh4-1 ( qui-1 ), shows a male sterile phenotype due to shortened filaments and pollenless anthers. a , b Inflorescences phenotypes of wild-type Col-0 ( a ) and qui-1 ( b ). Col-0 siliques are elongated and produce viable seeds, while mutant siliques fail to elongate and are devoid of any seeds. c , d Optical micrographs of Col-0 ( c ) and qui-1 ( d ) flowers. qui-1 develops stamens with filaments much shorter than Col-0. e – h Anthers of Col-0 ( e , g ) and qui-1 ( f , h ) visualized by a SEM microscope ( e , f ) and Alexander staining ( g , h ), respectively. Col-0 anthers give rise to viable pollen grains while mutant anthers are completely pollenless. Scale bars represent 1 cm in ( a ), ( b ), 0.5 mm in ( c ), ( d ), and 50 μm in ( e – h ) Full size image BES1 family members are essential for tapetum development To investigate the cellular basis causing pollen developmental defects, we made a series of semithin anther cross sections. We then compared the anatomical structures of anthers from Col-0 and qui-1 from stages 4–7 (Fig. 2 ). At stage 4 and early stage 5, the anther structures from Col-0 and qui-1 look indistinguishable (Fig. 2a, b, g, h ). The structural differences can be clearly observed from late stage 5, when the tapetum cells in Col-0 start to enlarge and differentiate (Fig. 2c ), cells at the same position remain unaltered in qui-1 (Fig. 2i ). Meanwhile, numbers of microsporocytes in qui-1 start to increase and partially crush the undeveloped tapetum-like cell layer (Fig. 2i ). At stage 6, Col-0 tapetum cells further enlarge and differentiate (Fig. 2d, e ), whereas tapetum-like cells in qui-1 fail to enlarge and differentiate (Fig. 2j, k ). At the meantime, the volume and cell numbers of microsporocytes are quickly increased in qui-1 but not in Col-0 (Fig. 2d, e, j, k ). At stage 7, Col-0 tapetum cells start to degenerate and tetrads are formed (Fig. 2f ). In qui-1 , microsporocytes cannot further develop into tetrads and cell death is initiated (Fig. 2l ). These observations indicated that the major reason causing the pollenless anthers in qui-1 is likely the abnormally developed tapetum. Fig. 2 qui-1 shows impaired tapetum differentiation and microsporogenesis starting from late stage 5. Semithin sections of anther lobes at different developmental stages from Col-0 ( a – f ) and qui-1 ( g – l ) after stained with toluidine blue. a , g Stage 4 anthers. The anthers from Col-0 and qui-1 showed no visible differences. b , h Early stage 5 anthers. The anthers from Col-0 and qui-1 showed no visible differences. c , i Late stage 5 anthers. Failed enlargement of tapetal cells and excessive microsporocytes were observed in qui-1 anthers. d , j Early stage 6 anthers. Significant excessive microsporocytes were observed in mutant anther locules. e , k Late stage 6 anthers. f , l Stage 7 anthers. Microsporocytes in qui-1 anthers cannot form tetrads. Epidermis (E), outer secondary parietal cell layer (OSP), inner secondary parietal cell layer (ISP), sporogenous cell (Sp), middle layer (ML), tapetum layer (T), tapetum-like layer (TL), microsporocytes (Ms), and tetrads (Tds) are indicated by arrows. Scale bars represent 20 μm Full size image To examine whether the tapetum-like cell layer in qui-1 losses tapetum cell identity, we carried out an in situ hybridization analysis to check the expression levels of two known tapetum marker genes, DYSFUNCTIONAL TAPETUM1 ( DYT1 ) [43] and ARABIDOPSIS THALIANA ANTHER 7 ( ATA7 ) [44] (Fig. 3a–f ). At stage 6 and stage 8, the expression of DYT1 and ATA7 can be, respectively, observed in the tapetum cell layer of Col-0 (Fig. 3a, d ). In qui-1 , however, the expression levels of these two genes are largely downregulated (Fig. 3b, e ). This result is consistent with the quantitative PCR analysis (Fig. 3g ). In addition, we also compared the expression levels of a number of tapetum identity related genes, including A6 [45] , A9 [46] , TDF1 [47] , AMS [48] , [49] , MS1 [50] , MS2 [51] , and MYB103 [52] , in Col-0 and qui-1 . In qui-1 , the expression levels of these selected genes are largely suppressed (Fig. 3g ). These data support our hypothesis that the tapetum cell identity in qui-1 has been altered. Fig. 3 BES1 family members are essential to tapetum development and function. a – f In situ hybridization analyses of DYT1 ( a – c ) and ATA7 ( d – f ) in the anthers of Col-0 ( a , d , c , f ) and qui-1 ( b , e ). Hybridization signals can be detected in stage 6 and stage 8 anthers of Col-0 ( a , d ), but not in the same-stage anthers of qui-1 ( b , e ), respectively. Sense probe was used as negative controls ( c , f ). Scale bars represent 20 μm. g Quantitative PCR analysis results to show relative expression levels of several tapetum marker genes in the inflorescences of Col-0 and qui-1 . Data are presented as mean and s.d. ( n = 3). Asterisks indicate significant differences ( P < 0.01, two-tailed t -test) Full size image BES1 and BZR1 are expressed in anthers If BES1, BZR1, and other family members are involved in the development of tapetum cells, they should be detected in the tapetum. To test this hypothesis, we successfully introduced pBES1::gBES1-YFP , pBZR1::gBZR1-YFP , pBEH1::gBEH1-YFP , and pBEH4::gBEH4-YFP into Col-0 and analyzed the localization of these proteins in anthers. Although they are not tapetum-specific proteins, tapetum localization of these four proteins can be clearly observed (Fig. 4 and Supplementary Fig. 5a–f ). Due to technical difficulties, we failed to clone pBEH2::gBEH2-YFP and pBEH3::gBEH3-YFP . To examine whether BEH2 and BEH3 are also expressed in the flowers, we generated transgenic plants carrying pBEH2::GUS or pBEH3::GUS and analyzed their expression patterns. Our GUS staining results indicated that both BEH2 and BEH3 are indeed expressed in the floral buds (Supplementary Fig. 5g–j ). The protein localization or gene expression results are consistent with our morphological analyses of qui-1 . Fig. 4 BES1-YFP and BZR1-YFP can be detected in the developing anthers. Seven-week-old pBES1::BES1-YFP ( a – f ) and pBZR1::BZR1-YFP ( g – l ) transgenic plants were used for confocal microscopic analyses. Stage 4–6 intact anthers were selected for analyzing the YFP signals. Green colors represent YFP signals and red colors are the auto-florescence of chlorophylls ( a – c , g – i ). To visualize detailed tissue-level localization of the YFP signal, somatic cell membranes were stained with FM4-64 ( d – f , j – l ). Inner secondary parietal cell layer (ISP) and tapetum (T) are indicated by arrow heads. Scale bars represent 20 μm Full size image The BES1 family acts independently of BR in tapetum development BES1 and BZR1 were thought to be the central regulators in the BR signal transduction, by mediating the expression of thousands of downstream BR response genes [20] , [21] , [26] , [27] . To investigate whether blocking the BR signaling pathway can cause similar tapetum defects as seen in qui-1 , we compared anthers from a BIN2 gain-of-function mutant, bin2-1 [16] , two null BRI1 mutants, bri1-701 [53] and bri1-116 [5] , a triple BR receptor mutant, bri1-701 brl1 brl3 , and a null mutant of a BR biosynthetic gene CPD , cpd [54] , with those from Col-0 and qui-1 by scanning electronic microscopy (Supplementary Fig. 6a ). Consistent with the results from a previous report [55] , all the BR-related mutants can produce pollen grains in their anthers, although they are only partially functional (Supplementary Fig. 6a ). qui-1 , on the other hand, cannot produce any pollen grains (Fig. 1e–h and Supplementary Fig. 6a ). Furthermore, we made semithin sections of anthers at different developmental stages for all aforementioned mutants and Col-0. As previously reported [55] , all the BR-related mutants contain a functional tapetum cell layer, although these cells are slightly more vacuolated (Supplementary Fig. 6b ). These data suggest BES1 family members have additional function besides their roles in regulating BR signaling. qui-2 anther phenotypes suggest link to TPD1-EMS1 signaling To investigate whether known tapetum regulatory components can regulate the activity of BES1 family members, we compared phenotypes of several published mutants with our quintuple mutants. We found that the defective anther phenotype of qui-1 is much closer to but slightly weaker than that of ems1 , tpd1 , and serk1 serk2 (Fig. 5a–d ). The major morphological difference is that ems1, tpd1, and serk1/2 completely lack a tapetum cell layer (Fig. 5d ), whereas qui-1 still has a tapetum-like cell layer (Fig. 5d ), although it lacks tapetum cell identity. Because qui-1 is leaky for BES1 and BEH4 , we generated additional mutants for BES1 and BEH4 , bes1-c1, bes1-c2, and beh4-c1 , by using CRISPR-Cas9. Sequence analyses indicated that bes1-c1 contains a consecutive 2-base pair (bp) mutation and two additional insertions of 8-bp and 24-bp, resulting in a premature stop codon (Supplementary Fig. 7 ). bes1-c2 and beh4-c1 contain 97-bp and 80-bp deletions, respectively (Supplementary Fig. 7 ). Because we did not obtain T-DNA insertion lines for BEH2 , we also generated a CRISPR-Cas9 mutant for BEH2 , beh2-c1 , in which a 28-bp deletion was identified by sequencing analysis (Supplementary Fig. 7 ). Therefore, the newly generated CRISPR-Cas9 mutants are considered null mutants. Using these new mutants and previous T-DNA null mutants for BZR1 , BEH1 , and BEH3 , we subsequently generated a second set quintuple mutant, bes1-c1 bzr1-1 beh1-1 beh3-1 beh4-c1 ( qui-2 ), a quadruple mutant, bes1-c1 bzr1-1 beh3-1 beh4-c1 ( qua-new ), and a sextuple mutant, bes1-c1 bzr1-1 beh1-1 beh2-c1 beh3-1 beh4-c1 . Similar to qui-1 , qui-2 does not contain any pollen grains and is completely male sterile (Fig. 5a–c and Supplementary Fig. 8 ). Semithin section analysis revealed that 60.2% anthers of qui-2 are identical to those of ems1 , tpd1 , and serk1/2 , in which the tapetum cell layer is absent (Fig. 5d and Supplementary Fig. 8h ). In qui-2 , 39.8% anthers only contain undifferentiated somatic cells, similar to those from spl (Supplementary Fig. 8l ). Unlike qui-1 , qui-2 shows a dwarfed stature (Supplementary Fig. 8a–d ), suggesting the BR signaling pathway has also been partially damaged. In bes1-c1 bzr1-1 beh1-1 beh2-c1 beh3-1 beh4-c1 sextuple mutant, 12.7% anthers contain 2–3 somatic cell layers surrounding the microsporocytes, and 87.3% anthers show a spl -like phenotype (Supplementary Fig. 8e, i, m ). Unsurprisingly, the tapetum defects of bes1-c1 bzr1-1 beh3-1 beh4-c1 is more severe than those of qui-1 but less severe than qui-2 (Supplementary Fig. 8f–h, j–l ). We also found the expression levels of tapetum marker genes, A6 , A9 , ATA7 , and DYT1 , are greatly downregulated in qui-1 , similar to those in ems1 , tpd1 , serk1/2 (Fig. 5e ). These genetic and molecular results strongly suggest BES1 family members act in the same signaling pathway with EMS1, TPD1, and SERK1/2 to control tapetum development. Fig. 5 bes1-1 bzr1-1 beh1-1 beh3-1 beh4-1 (qui-1) , bes1-c1 bzr1-1 beh1-1 beh3-1 beh4-c1 (qui-2) , tpd1 , serk1 serk2 , or ems1 show similar anther developmental defects. a Floral phenotypes of Col-0, qui-1 , qui-2 , tpd1 , serk1/2 , L er and ems1 . The qui-1 and qui-2 display shortened filaments similar to tpd1 , serk1 serk2 , and ems1 . b , c SEM microscopic ( b ) and Alexander staining ( c ) images of the anthers from the plants corresponding to ( a ). qui-1 and qui-2 anthers cannot produce pollen grains, reminiscent to those of tpd1 , serk1/2 , and ems1 . d Toluidine blue stained semithin sections of stage 6 anthers from plants corresponding to ( a ). All anthers of qui-1 , qui-2 , tpd1 , serk1/2 , and ems1 show excessive microsporocytes. qui-1 contains an impaired tapetal cell layer, whereas qui-2 only contains three somatic cell layers, lacking the tapetal cell layer, which is identical to those of tpd1 , serk1/2 , and ems1 . Number of somatic cell layers are indicated by red asterisks. e Quantitative RT-PCR results showing relative expression levels of tapetum marker genes in the inflorescences of various mutants and their corresponding wild-type backgrounds. Data are presented as mean and s.d. ( n = 3). Statistically significant differences between groups were tested using One-way ANOVA followed by LSD (least significant difference) post hoc test. Different letters indicate significant difference at P < 0.05. Scale bars represent 0.5 mm in ( a ), 50 μm in ( b ), ( c ), and 20 μm in ( d ) Full size image BES1 family members act downstream of TPD1-EMS1/SERK1/2 To confirm BES1 family members are in the same signaling pathway of TPD1-EMS1-SERK1/2, we introduced gain-of-function mutation of BES1 or BZR1 , bes1-D or bzr1-1D , into tpd1 , ems1 , and serk1/2 independently by genetic crossing (Fig. 6 and Supplementary Fig. 9 ). Genotypic and phenotypic analyses indicated the bes1-D and bzr1-1D can partially restore a functional tapetum cell layer, pollen development, and fertility in tpd1 , ems1 , and serk1/2 (Fig. 6 and Supplementary Fig. 9 ). bes1-D bzr1-1D double mutation showed better restoration to tpd1 than bes1-D or bzr1-1D single mutation (Fig. 6 ). Consistently, we found that the expression levels of several tapetum marker genes, A6 , A9 , ATA7 , and DYT1 , are greatly downregulated in tpd1 , and replacing BES1 with bes1-D , or BZR1 with bzr1-1D , or both BES1 and BZR1 with bes1-D and bzr1-1D , by genetic crossing can significantly recover the expression of these tapetum marker genes (Fig. 6p ). Different from their roles in tpd1 , ems1 , and serk1/2 , bes1-D and bzr1-1D cannot restore pollen development and fertility of dyt1 [43] , another mutant with defects in tapetum function (Supplementary Fig. 10 ). We also replaced BES1 or BZR1 with bes1-D or bzr1-1D in a number of other anther morphological mutants, including spl/nozzle [56] , [57] , bam1/2 [58] , and rpk2 [59] , no obvious fertility has been recovered (Supplementary Fig. 10 ). Our quantitative RT-PCR results indicated that the incapability of bes1-D or bzr1-1D to suppress the sterile phenotype of spl/nozzle , bam1/2 , and rpk1 is unlikely due to the low expression levels of bes1-D or bzr1-1D in these mutants (Supplementary Fig. 11 ). It is worth mentioning that 13.8% ( n = 80) lobes from spl bes1-D and 4.4% ( n = 68) lobes from spl bzr1-1D showed pollen-like structures by semithin section analyses, although both double mutants are still male sterile (Supplementary Fig. 12 ). These data indicated that the function of bes1-D and bzr1-1D in recovering the male reproduction defects of tpd1 , ems1 , and serk1/2 is mutant-specific. Fig. 6 bes1-D and bzr1-1D can partially suppress anther developmental defects and male sterility of tpd1 . a – e Toluidine blue stained anther semithin sections of Col-0 ( a ), tpd1 ( b ), tpd1 bes1-D ( c ), tpd1 bzr1-1D ( d ), and tpd1 bes1-D bzr1-1D ( e ). f – j Alexander stained anthers of Col-0 ( f ), tpd1 ( g ), tpd1 bes1-D ( h ), tpd1 bzr1-1D ( i ), and tpd1 bes1-D bzr1-1D ( j ). k – o Inflorescences of Col-0 ( k ), tpd1 ( l ), tpd1 bes1-D ( m ), tpd1 bzr1-1D ( n ), and tpd1 bes1-D bzr1-1D ( o ). Tapetum layer (T), and microsporocytes (Ms) are indicated by arrows. p Quantitative RT-PCR analyses to show relative gene expression levels of tapetum marker genes, A6 , A9 , ATA7 , and DYT1 in the inflorescences of Col-0, tpd1 , tpd1 bes1-D , tpd1 bzr1-1D , and tpd1 bes1-D bzr1-1D . Data are presented as mean and s.d. ( n = 3). Statistically significant differences between groups were tested using one-way ANOVA followed by LSD (least significant difference) post hoc test. Different letters indicate significant difference at P < 0.05. Scale bars represent 20 μm in ( a – e ), 50 μm in ( f – j ), and 1 cm in ( k – o ) Full size image If BES1 and its paralogs are the downstream components in TPD1-EMS1-SERK1/2 signaling pathway, we expect the activated ligand-receptor-co-receptor complex can activate BES1 and its paralogs. When BR signaling is initiated, non-phosphorylated BES1 can be greatly accumulated. We therefore tested whether similar consequence can occur. To exclude the interference of the BR signaling pathway, we also generated transgenic plants harboring pBRI1::TPD1 and pBRI1::EMS1-GFP in bri1-116 , individually. We then created double transgenic plants in Col-0 and in bri1-116 by genetic crossing. We tested the phosphorylation levels of BES1 with or without the treatment of brassinolide (BL), the final product of the BR biosynthetic pathway and the most active BR. Immunoblotting analysis indicated that without the treatment of BL, Col-0, TPD1 bri1-116 , and EMS1 bri1-116 showed very low levels of non-phosphorylated BES1 (Fig. 7a, b ). Interestingly, without exogenous treatment of BL, TPD1 EMS1-GFP bri1-116 , and TPD1 EMS1-GFP plants showed significant accumulation of non-phosphorylated BES1, reminiscent to that of BL-treated Col-0 (Fig. 7a, b ). Moreover, we compared the BES1-YFP and BZR1-YFP nuclear localization in Col-0 with those in ems1-c1 (a knockout mutant of EMS1 generated by using CRISPR-Cas9) (Supplementary Fig. 7 ), we found that the YFP signals are mainly localized in the tapetum cell nuclei in Col-0. But a significant amount of YFP signals can be detected in the cytoplasm of the somatic layer cells close to microsporocytes in ems1-c1 background, suggesting a functional EMS1 receptor is critical to the nuclear localization of BES1 and BZR1 (Fig. 7c, d ). These results demonstrate that BES1 not only can be activated by the BRI1-BR-BAK1 signaling pathway, but also by the EMS1-TPD1-SERK1/2 pathway, regardless of the BR signaling pathway. Fig. 7 BES1 can be activated by the EMS1-TPD1-SERK1/2 signaling pathway. a Immunoblotting analyses using transgenic plants harboring pBRI1::TPD1 ( TPD1 ), pBRI1::EMS1-GFP ( EMS1 ), or both in Col-0 indicated that the expression of TPD1 and EMS1 can lead to the accumulation of non-phosphorylated BES1. b The TPD1- and EMS1-induced accumulation of non-phosphorylated BES1 is independent of the BR signaling. Homemade anti-BES1 antibody was used to detect phosphorylated (p-BES1) or non-phosphorylated BES1 (BES1). bes1-c1 , bes1-c2 bzr1-c1 were used as negative controls for the anti-BES1 antibody. Coomassie Brilliant Blue stained rubisco protein was used as a loading control. EMS1-GFP and BRI1 immunoblotting analyses were carried out by using anti-GFP or anti-BRI1 antibody to confirm the accumulation of EMS1-GFP and the bri1-116 background, respectively. c , d Nuclear localization of BES1 or BZR1 in the somatic cell layer closest to the microsporocytes is partially dependent on the presence of EMS1. Scale bars represent 20 μm Full size image Our genetic, histological, molecular, and biochemical analyses demonstrate that BES1 family transcription factors play redundant and key roles in tapetum development. First, the bes1-1 bzr1-1 beh1-1 beh3-1 beh4-1 quintuple mutant ( qui-1 ) does not possess typical tapetum cell identity. At early stage 5 during anther development, the tapetum cell layer in qui-1 is indistinguishable from that in Col-0. The tapetal cells in qui-1 , however, cannot further expand at late stage 5 and are unable to stimulate the development of microsporocytes at the late anther developmental stages (Fig. 2 ). Tapetum marker genes and tapetum cell fate determination genes cannot be detected in these cell layers in qui-1 (Fig. 3 ). As a result, qui-1 microsporocytes fail to develop into functional pollen grains, causing male sterility (Fig. 1 and Supplementary Fig. 3 ). Although loss-of-function mutants of TPD1 , EMS1 , SERK1/2 , BES1 family members, and DYT1 show similar genetic consequence regarding microsporocyte development, their tapetum developmental defects are different. tpd1 , ems1 and serk1/2 lack tapetum cell layer, whereas qui-1 and dyt1 have a tapetum-like cell layer but they do not possess tapetum cell identity (Fig. 5 ). Why does qui-1 still contain a tapetum-like cell layer? One possibility is that there are still one fully functional BEH2 gene and partially functional BES1 and BEH4 in qui-1 . Alternatively, there could exist additional branching pathways besides the BES1-mediated pathway downstream of the EMS1-TPD1-SERK1/2 signaling to regulate the development of tapetum cell layer. To clarify these issues, we generated a number of null mutants for BES1 , BEH2 , and BEH4 by using a CRISPR-Cas9 approach and created the second set of quintuple mutant ( qui-2 ), and the sextuple mutant with all the BES1 family members being knocked out (Supplementary Figs. 7 , 8 ). A great portion of qui-2 lobes show only three somatic cell layers, identical to those from ems1 , tpd1 , and serk1/2 (Fig. 5d and Supplementary Fig. 8h ). The remaining portion of lobes exhibit spl -like phenotypes (Supplementary Fig. 8l ). In sextuple mutant, the majority lobes show a spl -like phenotype (Supplementary Fig. 8i, m ). These genetic results strongly suggest that the BES1 family members are in the same signaling pathway as EMS1-TPD1-SERK1/2. Second, our quantitative RT-PCR results indicated that all the tested downstream response genes for EMS1, are also the downstream response genes for BES1 family members (Fig. 5e ). Third, bes1-D and bzr1-1D can significantly suppress the male sterility of tpd1 , ems1 , and serk1/2 (Fig. 6 and Supplementary Fig. 9 ), but cannot restore that of dyt1 (Supplementary Fig. 10e, j, o, p ). Finally, the phosphorylation and nuclear localization of BES1 are regulated by EMS1-mediated pathway (Fig. 7 ). In summary, our data clearly demonstrate that BES1 family members are key downstream components of the EMS1-TPD1-SERK1/2 signaling cascade in controlling the differentiation and functions of tapetum (Fig. 8 ). Fig. 8 A current model showing that BES1 family members (or BES1 transcription factors, BES1 TFs) are essential downstream regulatory components in the TPD1-EMS1/SERKs pathway. In previous studies it was thought that BES1 family members play fundamental roles in regulating BR signaling pathway. A previous report proposed that EMS1 regulates tapetum development through interaction and activation of a group of beta carbonic anhydrases (β-CAs). In this study we suggest that BES1 family members can be activated by EMS1-mediated signaling to regulate tapetum formation. Our ChIP analyses suggest that BES1 and BZR1 can directly bind to the promoter regions of a number of tapetum developmental genes, such as SPL , DYT1 , and TDF1 . In addition, phenotypic similarity between the sextuple mutant and spl implies that BES1 family members may control SPL expression in earlier anther development. The detailed mechanism remains to be elucidated Full size image Given the fact that EMS1 , TPD1 , and SERK1/2 are all ubiquitously expressed [35] , [36] , [37] , [38] , [39] . If EMS1-TPD1-SERK1/2 can activate BR downstream transcription factor, BES1, why do BR signaling and biosynthetic mutants show an extremely severe defective phenotype? The activated BES1 from the EMS1-TPD1-SERK1/2 pathway should more or less compensate for the loss of the BR signaling pathway. One possible explanation is that in vegetative tissues, the EMS1-TPD1-SERK1/2 signaling pathway cannot be fully turned on due to under threshold concentrations of EMS1 and/or TPD1. Previous studies indicated that at early anther development stages (stages 2–5), the expression levels of EMS1 and TPD1 reach their peaks in anthers [35] , [36] , [37] . Possibly, only when EMS1 and TPD1 reach significant levels can the EMS1-TPD1-SERK1/2 signaling be initiated and the downstream signaling cascade be triggered, including the accumulation of non-phosphorylated BES1. Our quantitative RT-PCR results revealed that BRI1 is much less expressed than EMS1 in Arabidopsis inflorescences and siliques (Supplementary Fig. 13 ). In rosette leaves and cauline leaves, however, BRI1 is more expressed than EMS1 (Supplementary Fig. 13 ). Therefore, even though EMS1-TPD1-SERK1/2 and BRI1-BR-BAK1 share BES1 and its paralogs as their downstream signaling components, they may mainly function in separate territories, EMS1 functions predominantly in reproductive tissues and BRI1 plays a more significant role in the vegetative tissues. This notion is consistent with our biochemical results. For example, in Col-0 or bri1-116 , where EMS1-TPD1-SERK1/2 is present, non-phosphorylated BES1 was undetectable. But when EMS1 and TPD1 were both ectopically expressed in these plants by using a relatively stronger promoter, the BRI1 promoter, significant amount of non-phosphorylated BES1 can now be easily detected (Fig. 7 ). Interestingly, some of the 35S::EMS1 transgenic lines show significantly accumulated non-phosphorylated BES1 (Supplementary Fig. 14 ). While none of the 35S::TPD1 transgenic lines show significant accumulation of non-phosphorylated BES1 (Supplementary Fig. 14 ). In bri1 null mutants, plants are tiny, but anthers can still produce fairly normal pollen grains (Supplementary Fig. 6 ). In an ems1 null mutant, vegetative tissues look indistinguishable from those of wild-type Col-0, but tapetum development is greatly impaired. As a consequence, no pollen grains can be generated. Our genetic data suggest BES1 family members serve as downstream components of the EMS1-TPD1-SERK1/2 signaling complex and as upstream components of DYT1. For example, the expression levels of DYT1 in qui-1 is greatly reduced, and bes1-D or bzr1-1D cannot rescue the defective phenotypes of dyt1 (Fig. 3 and Supplementary Fig. 10 ). To test whether BES1 and BZR1 can directly regulate the expression of DYT1 , we carried out a chromatin immunoprecipitation (ChIP) analysis to investigate whether BES1 and BZR1 can be enriched in two E-box motifs within the DYT1 promoter region (Supplementary Fig. 15 ). As a matter of fact, BZR1 showed strong enrichment in both motifs. These data suggest BES1 family members may directly regulate the expression of DYT1 . Further detailed analyses are required to confirm such a conclusion. In addition, because a majority of anther lobes from sextuple mutant exhibit spl -like anther phenotypes, it is possible that BES1 family transcription factors may also regulate the expression of SPL in earlier anther development. As a matter of fact, a previous report indicated that BES1 can be enriched in the promoter region of SPL [55] . Our experiment also confirmed this result (Supplementary Fig. 15c ). Detailed analyses are also required to confirm such a scenario in the future. During our genetic analyses, we noticed that qui-2 and the sextuple mutant showed weak and strong bri1 phenotypes, respectively, confirming the significance of BES1 family members in regulating the BR signaling pathway. This report, however, focuses on the regulation of BES1 family members in tapetum development. Analyses of the genetic importance of BES1 family members in regulating the BR signaling pathway was discussed in a separate report [60] . Our data presented in this report contribute to a better understanding of the EMS1-TPD1-SERK1/2-mediated tapetum developmental signaling pathway, of which the downstream signaling components are largely uncharacterized. To our knowledge, this is also the first piece of evidence to show that BES1 family members can be shared by two distinctive RLK-mediated signaling pathways. It is likely that additional signaling pathways may also use BES1 family members as their downstream signaling components. Phylogenetic analysis Full-length amino acid sequences of BES1 family members were obtained from The Arabidopsis Information Resource (TAIR, https://www.arabidopsis.org/ ). Multiple sequence alignment was performed on MEGA 7.0.14 program ( https://www.megasoftware.net/home ) using MUSCLE method. The unrooted neighbor-joining phylogenetic tree was generated on the same program by using the Jones–Taylor–Thornton (JTT) model, and was gamma-distributed (gamma = 0.97) with 1000 bootstrap replicates. Plant materials and growth conditions The Arabidopsis thaliana Columbia (Col-0) and Landsberg erecta (L er ) ecotypes were used in this study. Mutants of BES1 and its paralogs were obtained from ABRC with accession numbers: bes1-1 (SALK_098634), bzr1-1 (GK_857E04), beh1-1 (GK_432C09), beh3-1 (SALK_017577), beh4-1 (SALK_055421). 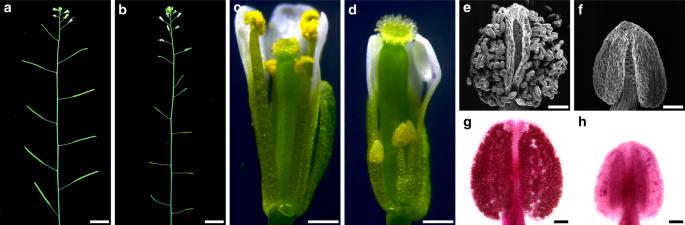Fig. 1 A quintuple mutant,bes1-1 bzr1-1 beh1-1 beh3-1 beh4-1(qui-1), shows a male sterile phenotype due to shortened filaments and pollenless anthers.a,bInflorescences phenotypes of wild-type Col-0 (a) andqui-1(b). Col-0 siliques are elongated and produce viable seeds, while mutant siliques fail to elongate and are devoid of any seeds.c,dOptical micrographs of Col-0 (c) andqui-1(d) flowers.qui-1develops stamens with filaments much shorter than Col-0.e–hAnthers of Col-0 (e,g) andqui-1(f,h) visualized by a SEM microscope (e,f) and Alexander staining (g,h), respectively. Col-0 anthers give rise to viable pollen grains while mutant anthers are completely pollenless. Scale bars represent 1 cm in (a), (b), 0.5 mm in (c), (d), and 50 μm in (e–h) Primers for genotyping are listed in Supplementary Table 1 . The other Arabidopsis lines are described previously: bri1-701 [53] , bri1-116 [5] , serk1/2 [53] , cpd [54] , bin2-1 [16] , bes1-D [21] , bzr1-1D [20] , tpd1 [37] , ems1 [36] , bam1/2 [58] , spl [57] , rpk2 [59] , and dyt1 [43] . After vernalizing at 4 °C for 2 days, all the described wild-type and mutant seeds were planted and grown in soil at 22 °C under 16 h-light/8 h-dark photoperiod condition. For western blot analysis, seeds were grown on half-strength Murashige and Skoog (1/2 MS) agar plates, supplemented with 1% (w/v) sucrose under the same condition described above. Generation of constructs and transgenic plants For complementation, promoter (~1.5 kb) plus genomic sequences of BES1 and its paralogs (except BEH3 ) were cloned into a Gateway™ Entry vector, then subcloned into a binary destination vector pBIB-BASTA-GWR. Coding sequence of BEH3 was cloned into the Gateway entry vector, then subcloned into a pBIB-BASTA-pUBQ10-GWR vector, derived from a pBIB-BASTA-35S-GWR binary vector. For expression analysis, the entry vectors of BES1 and its paralogs were subcloned into a pBIB-BASTA-GWR-YFP destination vector. For ectopic expression, coding sequences of EMS1 and TPD1 were cloned into entry vector and then subcloned into pBIB-BASTA-35S-GWR, pBIB-KAN-pBRI1-GWR-GFP, and pBIB-HYG-pBRI1-GWR vectors, respectively. The constructs were then transformed into Col-0, bri1-116 +/− , and quintuple mutants through the floral dip method [61] . Photographing and microscopy For phenotypic observation, photos of 7-week inflorescences of all genotypes were taken with a Canon EOS 70D Camera. Pictures of flowers from each genotype were taken with a Leica M165C Stereomicroscope. For scanning microscopic analyses, anthers were removed from fully opened flowers and carefully set on the sample preparation platform and quickly frozen in liquid nitrogen, the samples were then immediately transferred into the chamber of a Hitachi S-3400N scanning electron microscope before the images were taken. For pollen viability analysis, flower buds at development stage 12 were fixed with Carnoy’s fixative containing 60% ethanol, 30% chloroform, and 10% acetic acid for at least 2 h. Individual anthers were obtained and stained with Alexander’s solution for 30 min at 25 °C, the anthers were visualized and photographed with a Leica DM6000 B microscope. For anatomic studies of anthers, entire inflorescences were fixed in FAA fixative and dehydrated with a series of graded ethanol. After dehydration, the inflorescences were embedded in Technovit 7100 resin. Cross sections were made by a rotary microtome with thickness of 2 μm. The sections were then stained with 0.5% toluidine blue and the images were taken using a Leica DM6000 B microscope. For expression pattern analyses of YFP inframe-fused BES1 and its paralogs, anthers from stages 4–6 were mounted in water and were observed under a Leica TCS SP8 laser scanning confocal microscope. YFP and chlorophyll signals were excited at a 514-nm laser wave length. The emission was captured using PMTs set at 517–543 and 620–690 nm, respectively. In addition, for tapetum localization of BES1, anthers were mounted and stained on slides with FM4-64 solution for at least 30 min before visualizing and photographing. YFP signal was excited and captured as described. The FM4-64 signal was excited at a 514-nm laser wave length and captured with PTM set at 620–680 nm. RT-PCR and qRT-PCR RT-PCR was used to determine the target gene expression in mutants and transgenic plants. qRT-PCR was used to evaluate the expression levels of genes that either function in or used as markers during anther development. Total RNAs were extracted from rosette leaves (RT-PCR) and inflorescences before stage 12 (qRT-PCR) using an RNAsimple Total RNA Kit (TIANGEN). cDNA was generated with the PrimeScript™ 1st Strand cDNA Synthesis Kit (Takara). For RT-PCR, genes were amplified from 100 ng total RNA reverse transcripts. For qRT-PCR, genes were amplified from 40 ng total RNA reverse transcripts. All primers used are listed in Supplementary Table 1 . SYBR Premix Ex Taq II (Takara) was used in PCR reaction on a StepOnePlus Real-Time PCR System (Applied Biosystems™). All experiments were performed in triplicate. RNA in situ hybridization Inflorescences were fixed with ice-cold 4% (w/v) paraformaldehyde in glass vials on ice. After fixation in vacuum ambiance, samples were dehydrated in a series of graded ethanol. Fully dehydrated samples were stained with Eosin Y in absolute ethanol and then were cleared with graded Histo-clear/ethanol solutions. When the ethanol was replaced by pure Histo-clear, the samples were transferred into a 60 °C oven and the Histo-clear was gradually infiltrated with Paraplast (Leica). Then the fully infiltrated samples were embedded into Paraplast for sectioning. Eight-micrometer-thick cross sections on slides were dewaxed and treated with proteinase K. In vitro RNA probe synthesis, hybridization and signal detection were performed according to the manual of the DIG RNA labeling kit (Roche; 11175025910). Primers used were listed in Supplementary Table 1 . Images were taken by using a Leica DM6000 B microscope. Western blot analysis After genotyping, 2-week-old double transgenic plants in bri1-116 background were treated with or without 100 nM BL (Sigma) for 90 min. Total proteins were extracted with 2 × SDS buffer containing 125 mM Tris (pH 6.8), 4% (w/v) SDS, 20% (v/v) glycerol, 20 mM DTT, 0.02% (w/v) bromophenol blue. Protein extracts equivalent to 7.5 mg seedlings were resolved on 7% (for GFP and BRI1) and 11% (for BES1) Bis-Tris SDS-PAGE gel and transferred onto a nitrocellulose membrane. After blocking with 5% milk solution, the membranes were incubated with primary antibodies against GFP (1:3000, Roche, 11814460001), BRI1 (1:2000, Agrisera, AS121859), and BES1 (1:5000, homemade), respectively, and then the corresponding HRP-conjugated secondary antibodies (1:5000, Abmart, anti-mouse (M21001) for GFP, and anti-rabbit (M21002) for BES1 and BRI1). The signals were revealed by a JustGene ECL Plus (CLINX) mixture and were detected by a Tanon 5200 chemiluminescence image analysis system. CRISPR/Cas9 All CRISPR/Cas9 mutants mentioned were generated by using the egg cell-specific promoter-controlled (EPC) CRISPR/Cas9 system as previously reported [62] , [63] . For these genes, Target 1-(gRNA-Sc)-(U6-26t)-(U6-29p)-Target 2 were amplified from a pCBC-DT1T2 vector template by using the primers including the sgRNA sequence. The PCR fragments were transformed into a pHEE401E binary vector through a restriction–ligation method. The constructs were then transformed into corresponding Arabidopsis genotypes using Agrobacterium -mediated floral dip method [61] . The transgenic lines were confirmed by PCR and sequencing, and were crossed with their backgrounds for separation of the vector. 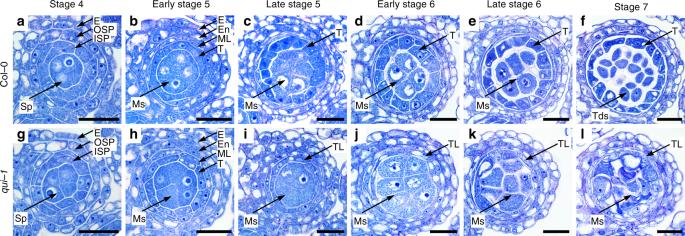Fig. 2 qui-1shows impaired tapetum differentiation and microsporogenesis starting from late stage 5. Semithin sections of anther lobes at different developmental stages from Col-0 (a–f) andqui-1(g–l) after stained with toluidine blue.a,gStage 4 anthers. The anthers from Col-0 andqui-1showed no visible differences.b,hEarly stage 5 anthers. The anthers from Col-0 andqui-1showed no visible differences.c,iLate stage 5 anthers. Failed enlargement of tapetal cells and excessive microsporocytes were observed inqui-1anthers.d,jEarly stage 6 anthers. Significant excessive microsporocytes were observed in mutant anther locules.e,kLate stage 6 anthers.f,lStage 7 anthers. Microsporocytes inqui-1anthers cannot form tetrads. Epidermis (E), outer secondary parietal cell layer (OSP), inner secondary parietal cell layer (ISP), sporogenous cell (Sp), middle layer (ML), tapetum layer (T), tapetum-like layer (TL), microsporocytes (Ms), and tetrads (Tds) are indicated by arrows. Scale bars represent 20 μm The sequence information of targets and primers is listed in Supplementary Table 2 . ChIP assay Chromatin immunoprecipitation was performed according to a previous report with minor modifications [64] . Briefly, 2 g inflorescence materials from 6-week-old Col-0, pBES1::BES1-YFP , and pBZR1::BZR1-YFP plants were cross-linked in sucrose-formaldehyde buffer (0.4 M sucrose, 10 mM Tris-HCl (pH 8), 1 mM PMSF, 1 mM EDTA, 1% formaldehyde). Nuclei were isolated with nuclei isolation buffer (0.25 M sucrose, 15 mM PIPES (pH 6.8), 5 mM MgCl 2 , 60 mM KCl, 15 mM NaCl, 1 mM CaCl 2 , 0.9% Triton X-100, 1 ×proteinase inhibitor) and then were lysed with lysis buffer (50 mM HEPES (pH 7.5), 150 mM NaCl, 1 mM EDTA, 1 mM PMSF, 1% SDS, 0.1% Na deoxycholate, 1% Triton X-100, 1 × proteinase inhibitor). The lysates were sonicated to generate DNA fragments with an average size of 500 bp. After 10-times dilution with dilution buffer (50 mM HEPES (pH 7.5), 150 mM NaCl, 1 mM EDTA, 1 mM PMSF, 0.1% Na deoxycholate, 0.4% Triton X-100, 1 × proteinase inhibitor), the solubilized chromatin was immunoprecipitated by an agarose-conjugated anti-GFP antibody. The coimmunoprecipitated DNA was analyzed by quantitative PCR as described above. The primers are listed in Supplementary Table 1 . Statistical analysis All values are presented as mean and standard deviation (s.d.). The significance of differences for pairwise comparisons was estimated by two-tailed student’s t -tests. The statistical significance of differences between groups were compared on SPSS statistics program using one-way ANOVA followed by least significant difference post hoc test at P < 0.05. 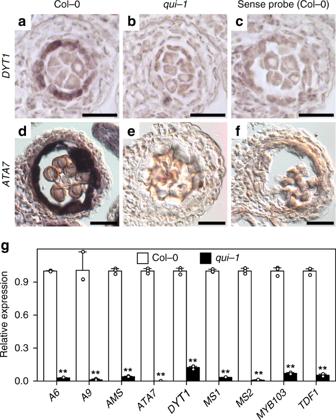Fig. 3 BES1 family members are essential to tapetum development and function.a–fIn situ hybridization analyses ofDYT1(a–c) andATA7(d–f) in the anthers of Col-0 (a,d,c,f) andqui-1(b,e). Hybridization signals can be detected in stage 6 and stage 8 anthers of Col-0 (a,d), but not in the same-stage anthers ofqui-1(b,e), respectively. Sense probe was used as negative controls (c,f). Scale bars represent 20 μm.gQuantitative PCR analysis results to show relative expression levels of several tapetum marker genes in the inflorescences of Col-0 andqui-1. Data are presented as mean and s.d. (n= 3). Asterisks indicate significant differences (P< 0.01, two-tailedt-test) 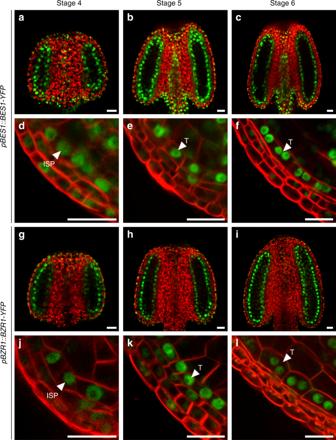Fig. 4 BES1-YFP and BZR1-YFP can be detected in the developing anthers. Seven-week-oldpBES1::BES1-YFP(a–f) andpBZR1::BZR1-YFP(g–l) transgenic plants were used for confocal microscopic analyses. Stage 4–6 intact anthers were selected for analyzing the YFP signals. Green colors represent YFP signals and red colors are the auto-florescence of chlorophylls (a–c,g–i). To visualize detailed tissue-level localization of the YFP signal, somatic cell membranes were stained with FM4-64 (d–f,j–l). Inner secondary parietal cell layer (ISP) and tapetum (T) are indicated by arrow heads. Scale bars represent 20 μm 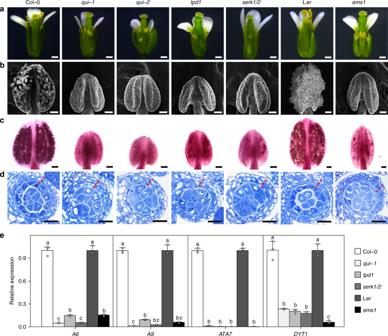Fig. 5 bes1-1 bzr1-1 beh1-1 beh3-1 beh4-1 (qui-1),bes1-c1 bzr1-1 beh1-1 beh3-1 beh4-c1 (qui-2),tpd1,serk1 serk2, orems1show similar anther developmental defects.aFloral phenotypes of Col-0,qui-1,qui-2,tpd1,serk1/2, Lerandems1. Thequi-1andqui-2display shortened filaments similar totpd1,serk1 serk2, andems1.b,cSEM microscopic (b) and Alexander staining (c) images of the anthers from the plants corresponding to (a).qui-1andqui-2anthers cannot produce pollen grains, reminiscent to those oftpd1,serk1/2, andems1.dToluidine blue stained semithin sections of stage 6 anthers from plants corresponding to (a). All anthers ofqui-1,qui-2,tpd1,serk1/2, andems1show excessive microsporocytes.qui-1contains an impaired tapetal cell layer, whereasqui-2only contains three somatic cell layers, lacking the tapetal cell layer, which is identical to those oftpd1,serk1/2, andems1. Number of somatic cell layers are indicated by red asterisks.eQuantitative RT-PCR results showing relative expression levels of tapetum marker genes in the inflorescences of various mutants and their corresponding wild-type backgrounds. Data are presented as mean and s.d. (n= 3). Statistically significant differences between groups were tested using One-way ANOVA followed by LSD (least significant difference) post hoc test. Different letters indicate significant difference atP< 0.05. Scale bars represent 0.5 mm in (a), 50 μm in (b), (c), and 20 μm in (d) 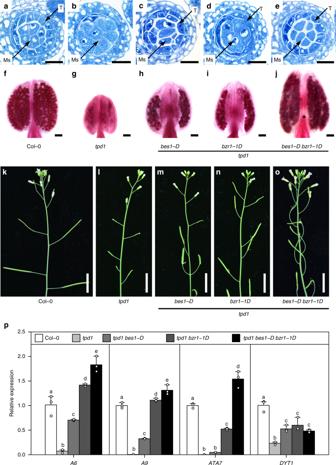Fig. 6 bes1-Dandbzr1-1Dcan partially suppress anther developmental defects and male sterility oftpd1.a–eToluidine blue stained anther semithin sections of Col-0 (a),tpd1(b),tpd1 bes1-D(c),tpd1 bzr1-1D(d), andtpd1 bes1-D bzr1-1D(e).f–jAlexander stained anthers of Col-0 (f),tpd1(g),tpd1 bes1-D(h),tpd1 bzr1-1D(i), andtpd1 bes1-D bzr1-1D(j).k–oInflorescences of Col-0 (k),tpd1(l),tpd1 bes1-D(m),tpd1 bzr1-1D(n), andtpd1 bes1-D bzr1-1D(o). Tapetum layer (T), and microsporocytes (Ms) are indicated by arrows.pQuantitative RT-PCR analyses to show relative gene expression levels of tapetum marker genes,A6,A9,ATA7, andDYT1in the inflorescences of Col-0,tpd1,tpd1 bes1-D,tpd1 bzr1-1D, andtpd1 bes1-D bzr1-1D. Data are presented as mean and s.d. (n= 3). Statistically significant differences between groups were tested using one-way ANOVA followed by LSD (least significant difference) post hoc test. Different letters indicate significant difference atP< 0.05. Scale bars represent 20 μm in (a–e), 50 μm in (f–j), and 1 cm in (k–o) 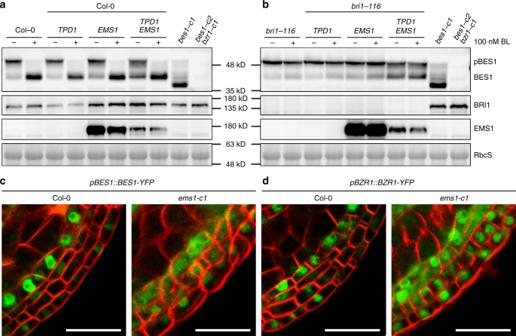Fig. 7 BES1 can be activated by the EMS1-TPD1-SERK1/2 signaling pathway.aImmunoblotting analyses using transgenic plants harboringpBRI1::TPD1(TPD1),pBRI1::EMS1-GFP(EMS1), or both in Col-0 indicated that the expression ofTPD1andEMS1can lead to the accumulation of non-phosphorylated BES1.bThe TPD1- and EMS1-induced accumulation of non-phosphorylated BES1 is independent of the BR signaling. Homemade anti-BES1 antibody was used to detect phosphorylated (p-BES1) or non-phosphorylated BES1 (BES1).bes1-c1,bes1-c2 bzr1-c1were used as negative controls for the anti-BES1 antibody. Coomassie Brilliant Blue stained rubisco protein was used as a loading control. EMS1-GFP and BRI1 immunoblotting analyses were carried out by using anti-GFP or anti-BRI1 antibody to confirm the accumulation of EMS1-GFP and thebri1-116background, respectively.c,dNuclear localization of BES1 or BZR1 in the somatic cell layer closest to the microsporocytes is partially dependent on the presence of EMS1. Scale bars represent 20 μm 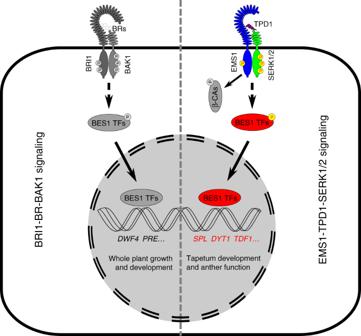Fig. 8 A current model showing that BES1 family members (or BES1 transcription factors, BES1 TFs) are essential downstream regulatory components in the TPD1-EMS1/SERKs pathway. In previous studies it was thought that BES1 family members play fundamental roles in regulating BR signaling pathway. A previous report proposed that EMS1 regulates tapetum development through interaction and activation of a group of beta carbonic anhydrases (β-CAs). In this study we suggest that BES1 family members can be activated by EMS1-mediated signaling to regulate tapetum formation. Our ChIP analyses suggest that BES1 and BZR1 can directly bind to the promoter regions of a number of tapetum developmental genes, such asSPL,DYT1, andTDF1. In addition, phenotypic similarity between the sextuple mutant andsplimplies that BES1 family members may controlSPLexpression in earlier anther development. The detailed mechanism remains to be elucidated Reporting summary Further information on research design is available in the Nature Research Reporting Summary linked to this article.